Population decline is linked to migration route in the Common Cuckoo Migratory species are in rapid decline globally. Although most mortality in long-distance migrant birds is thought to occur during migration, evidence of conditions on migration affecting breeding population sizes has been completely lacking. We addressed this by tracking 42 male Common Cuckoos from the rapidly declining UK population during 56 autumn migrations in 2011–14. Uniquely, the birds use two distinct routes to reach the same wintering grounds, allowing assessment of survival during migration independently of origin and destination. Mortality up to completion of the Sahara crossing (the major ecological barrier encountered in both routes) is higher for birds using the shorter route. The proportion of birds using this route strongly correlates with population decline across nine local breeding populations. Knowledge of variability in migratory behaviour and performance linked to robust population change data may therefore be necessary to understand population declines of migratory species and efficiently target conservation resources. Migratory species are increasingly threatened across the globe [1] driven by climate change [2] , [3] , habitat change and habitat loss [4] , [5] . Understanding where mortality occurs during their annual cycles is therefore increasingly important, especially for organisms such as long-distance migrant land birds, which show some of the steepest population declines [4] , [5] . The breeding behaviour of one such species considered here, the obligate brood parasite Common Cuckoo, has been extremely well studied but its migration routes have been very poorly known until now [6] . As migration periods have been implicated as the stage of the annual cycle during which most mortality occurs in migrants [7] , [8] , understanding the variability of migration routes and associated patterns of mortality in these birds is vital to untangling the causes of their population declines. Until very recently, most migratory birds have, however, been too small to carry the tracking devices that have been available. Consequently, study of their seasonal mortality and migration routes has so far been restricted to indirect [7] and strongly biased [9] methods, and evidence of migration mortality impacting on breeding populations has been lacking, despite its potential to do so [10] . Miniaturization of archival light-level recorders, known as ‘geolocators’ [11] , has recently allowed us to re-construct the migratory paths of some smaller species, providing insight into their migration strategies [12] and how environmental conditions can constrain them [13] . However, as data are restricted to individuals that successfully return to allow data retrieval, these devices do not allow the study of patterns of mortality. Recent availability of platform transmitter terminals (PTTs) as small as 5 g, however, has enabled us to track the migrations and mortality of the largest nocturnally migrating long-distance migrant land birds, such as Common Cuckoos, in close to real time [14] . Detailed monitoring of breeding birds in the United Kingdom [15] , [16] has shown that this species population is rapidly declining, but that population trends vary locally. This enabled us to track birds from widely spaced localities with a range of cuckoo population trajectories, to test whether there is a relationship between migratory behaviour and the degree of local population change. We found that the birds used two distinct routes to reach the same wintering grounds, allowing assessment of survival during migration independent of origin and destination. Mortality up to completion of the Sahara crossing (the major ecological barrier encountered in both routes) was higher for birds using the route that was shorter up to that point. The proportion of birds using this route strongly correlated with population decline across nine local breeding populations. These results demonstrate that mortality during migration can impact breeding populations of long-distance migrants. Consequently, knowledge of variability in migratory behaviour and performance linked to robust population change data may be necessary to understand population declines of migratory species and to efficiently target conservation resources. Migration routes and survival We tracked cuckoos from nine widely spaced localities within the United Kingdom, which varied in major habitat type and probably cuckoo host species, as well as cuckoo population trajectories. Two localities were in the Highlands of Scotland (Kinloch & Skye and Trossachs National Park), one in the uplands of central Wales (Tregaron), three across the south of England (Dartmoor, New Forest and Ashdown Forest), one in the East Midlands (Sherwood Forest) and two in East Anglia (Thetford Forest and Norfolk Broads) ( Fig. 1 and Supplementary Tables 1 and 2 ). The birds used two distinct routes during migration from the United Kingdom, heading either Southwest (West route) via Spain or Southeast (East route) via Italy or the Balkans ( Fig. 2a ), with very high individual route consistency between years ( Supplementary Fig. 1 ). However, all used the same Central African wintering grounds ( Fig. 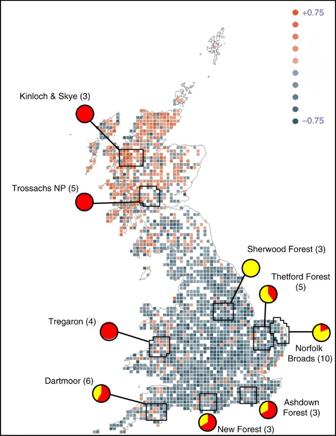Figure 1: Cuckoo migration route use and breeding population change for each tagging location. Population change is shown at 10 km2resolution. For each tagging location, pie charts show the proportion of tagged birds that migrated East (red) and West (yellow) (sample size of birds is given in parentheses after each tagging location name) and black polygons outline the 10 km2area that contributed to the population change index (see Methods andSupplementary Tables 1 and 2). Colour of 10 km2indicates the proportional population change between the BTO Atlases in 1988–91 and 2007–11 according to the scheme shown in the figure, with dark pink indicating the largest increase, dark grey the largest decrease and white indicating no change15. 2a,b and Table 1 ). As local breeding populations varied strongly in their composition of West and East migrating individuals ( Fig. 1 ), we were able to assess differences in mortality associated with the two migration routes, while controlling for both area of origin and destination. Figure 1: Cuckoo migration route use and breeding population change for each tagging location. Population change is shown at 10 km 2 resolution. For each tagging location, pie charts show the proportion of tagged birds that migrated East (red) and West (yellow) (sample size of birds is given in parentheses after each tagging location name) and black polygons outline the 10 km 2 area that contributed to the population change index (see Methods and Supplementary Tables 1 and 2 ). Colour of 10 km 2 indicates the proportional population change between the BTO Atlases in 1988–91 and 2007–11 according to the scheme shown in the figure, with dark pink indicating the largest increase, dark grey the largest decrease and white indicating no change [15] . 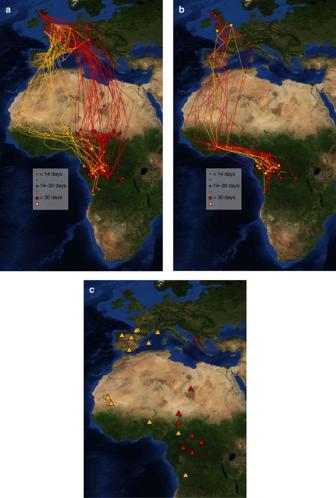Figure 2: Migration routes and apparent mortality locations of tagged cuckoos. (a) Autumn (southwards) and (b) spring (northwards) migration routes and stopover locations, and (c) apparent mortality locations during autumn migration of cuckoos using the East (red) and West (yellow) routes. Ina,b, circle size indicates stopover duration as shown in the key. There was no difference in the final (mid-winter) locations of birds using the two routes (binomial GLMM; latitude: df 1, 7, F=1.09,P=0.332; longitude: df 1, 7, F=0,P=0.962; latitude*longitude: df 1, 7, F=1.3,P=0.292). Estimates of survival of birds using the two routes are given in the text. Base map OpenStreetMap contributors. Full size image Figure 2: Migration routes and apparent mortality locations of tagged cuckoos. ( a ) Autumn (southwards) and ( b ) spring (northwards) migration routes and stopover locations, and ( c ) apparent mortality locations during autumn migration of cuckoos using the East (red) and West (yellow) routes. In a , b , circle size indicates stopover duration as shown in the key. There was no difference in the final (mid-winter) locations of birds using the two routes (binomial GLMM; latitude: df 1, 7, F=1.09, P =0.332; longitude: df 1, 7, F=0, P =0.962; latitude*longitude: df 1, 7, F=1.3, P =0.292). Estimates of survival of birds using the two routes are given in the text. Base map OpenStreetMap contributors. Full size image Table 1 Comparison of migrations through the Western and Eastern routes. Full size table Estimated apparent survival rates across both routes were 0.799 (95% confidence limits 0.615–0.908) up to completion of the Sahara crossing, 0.776 (95% confidence limits 0.604–0.807) during remainder of autumn migration and 0.675 (95% confidence limits 0.448–0.841) from completion of autumn migration up to return to the United Kingdom. Up to completion of the Sahara crossing, the survival of birds taking the West route was lower than that of bird taking the East route (binomial generalised linear mixed model (GLMM); df 1, 10, F=7.96, P =0.018; estimates: East: 0.976, 95% confidence limits 0.673–0.999; West: 0.562, 95% confidence limits 0.106–0.928) based on 33 migrations by 22 individuals taking the East route and 23 migrations by 20 individuals taking the West route. When including only the first journey from each individual, the result was very similar (binomial GLMM; df 1, 30, F=6.66, P =0.015; East: 0.956, 95% confidence limits 0.677–0.996; West 0.538, 95% confidence limits 0.163–0.875). There was no difference in survival during the remainder of autumn migration (binomial GLMM; df 1, 9, F=0.02, P =0.904) (East: 31 migrations by 20 birds, West: 14 migrations by 13 birds) or from completion of autumn migration up to return to the United Kingdom (binomial GLMM; df 1, 6, F=1.52, P =0.263), but sample size was small for the latter (East: 24 migrations by 16 birds, West: 11 migrations by 10 birds). Excluding cases most likely to be tag failure (see Methods) resulted in the removal of one bird from both East and West routes for autumn migration up to completion of the Sahara crossing and the survival of birds taking the West route was still lower than for those taking the East route (binomial GLMM; df 1, 10, F=7.72, P =0.019; estimates: East 0.985, 95% confidence limits 0.730–0.999; West 0.596, 95% confidence limits 0.144–0.928). After the removal of one bird from the East route for the remainder of autumn migration, there was still no difference in apparent survival between the routes (binomial GLMM; df 1, 9, F=0.01, P =0.938; estimates: East 0.797, 95% confidence limits 0.573–0.920; West 0.786, 95% confidence limits 0.447–0.944). No cases were removed for the period from arrival at the midwinter location up to return to the United Kingdom. Survival to completion of the Sahara crossing, the major ecological barrier encountered in both migration routes, was therefore significantly lower in the West route, which is 12% shorter to that point ( Table 1 ), whereas there was no difference in apparent survival during the remainder of their migrations through tropical Africa. This demonstrates that the costs of migration may be route specific and are not necessarily related directly to migration distance. Migration routes and local population change Across the nine areas of the United Kingdom in which cuckoos were tagged, the proportion of birds using the West route, associated with lower survival, was correlated with the degree of local breeding population decline assessed using two independent population change data sets—national breeding bird Atlases in 1998–2001 and 2007–11 (ref. 15 ), and the annual Breeding Bird Survey (BBS) [16] ( Fig. 3 ). Although there was some geographical association of the routes within Britain, with all birds from the upland areas in Scotland and Wales using the East route, the correlation between route use and population change remained for the more robust change data set (see Fig. 3 legend) from the Atlases after controlling for the upland/lowland division ( Fig. 3 ). This provides the first direct evidence that conditions encountered during migration can have an impact on breeding populations. 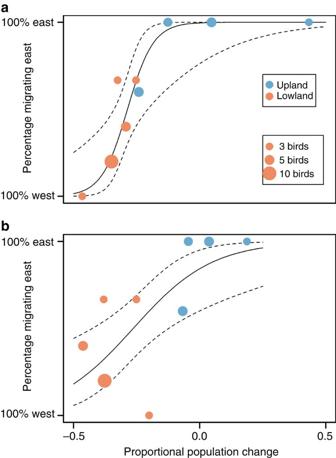Figure 3: Relationship between migration route use and population change across nine tagging locations. Results are shown for (a) Atlas and (b) BBS cuckoo population change data sets and are based on events/trials logistic regressions where the migration directions of individual birds tagged in each locality are predicted by population change variables (see Methods). The modelled effect of migration route is shown by the solid line and its 95% confidence intervals by the dotted lines. The relationship was highly significant for both data sets (events/trials logistic regression; Atlas: df 1,χ222.7, P<0.0001; BBS: df 1,χ212.0,P=0.0005). When controlling for the upland/lowland habitat division (see Methods for definition), the relationship remained highly significant for the Atlas data set events/trials logistic regression; (df 1,χ28.7,P<0.0031) but not for the BBS data set (events/trials logistic regression; df 1,χ20.0,P=0.842). Atlas population change data are from surveys of 39,936 2 km2in 1998–91 and 45,374 in 2007–11. BBS data set population change was based on surveys of up to 3,018 1 km2each year between 1994–96 and 2007–11, requiring interpolation to give national coverage, and is therefore less robust for assessing local population changes. Habitat classification, migration route and population change data for each tagging location are shown inSupplementary Table 2. Figure 3: Relationship between migration route use and population change across nine tagging locations. Results are shown for ( a ) Atlas and ( b ) BBS cuckoo population change data sets and are based on events/trials logistic regressions where the migration directions of individual birds tagged in each locality are predicted by population change variables (see Methods). The modelled effect of migration route is shown by the solid line and its 95% confidence intervals by the dotted lines. The relationship was highly significant for both data sets (events/trials logistic regression; Atlas: df 1, χ 2 22.7, P<0.0001; BBS: df 1, χ 2 12.0, P =0.0005). When controlling for the upland/lowland habitat division (see Methods for definition), the relationship remained highly significant for the Atlas data set events/trials logistic regression; (df 1, χ 2 8.7, P <0.0031) but not for the BBS data set (events/trials logistic regression; df 1, χ 2 0.0, P =0.842). Atlas population change data are from surveys of 39,936 2 km 2 in 1998–91 and 45,374 in 2007–11. BBS data set population change was based on surveys of up to 3,018 1 km 2 each year between 1994–96 and 2007–11, requiring interpolation to give national coverage, and is therefore less robust for assessing local population changes. Habitat classification, migration route and population change data for each tagging location are shown in Supplementary Table 2 . Full size image Potential drivers of mortality Unexpectedly [7] , most of the excess mortality associated with the West route occurred in Europe, before the desert crossing ( Fig. 2c ). It is therefore likely to be that conditions at stopovers in this area are responsible. Decreasing rainfall in Spain [17] is a possible cause. Increasingly severe droughts and associated wildfires have occurred in recent years, for example, in 2012, when none of three birds taking the West route survived to complete the desert crossing. Other possibilities include large-scale habitat changes or increased predation pressure. Migration strategies are thought to be more energy-selected in autumn compared with spring when they are time selected [18] ; thus, autumn migration strategies are likely to have evolved in relation to energy availability at stopovers, making them vulnerable to the effects of environmental change at this time. Birds using the West route left the breeding grounds on average 8 days later and subsequently spent less time in stopovers before crossing the Sahara than birds using the East route ( Table 1 ), possibly undertaking more pre-migratory fattening at the breeding location. Changing conditions on the breeding grounds, such as the declines of the large moths whose caterpillars are the major food source for adult cuckoos, which have been particularly severe in the areas in which birds using the West strategy were tagged [19] , may therefore have an impact on them more than birds taking the East route and would exacerbate the effects of poor conditions on stopovers further south in Europe. A larger sample of individuals and years is, however, required to determine the potentially interactive effects of conditions in both the United Kingdom and on stopovers in mainland Europe on survival of cuckoos using the two routes. Origin and persistence of the two migration routes The presence of birds within the Unitd Kingdom using two distinct routes to reach the same wintering grounds provided a unique opportunity to assess survival on migration independently of origin and destination. Double colonization after the last ice age by birds with different evolutionary histories, including migration routes, is a probable explanation for the occurrence within England of birds using two different routes. Genetic analysis is required, however, to determine whether England is in fact such a secondary contact zone [20] , although there is some evidence that birds from adjacent parts of mainland Europe, such as Belgium where the population of Common Cuckoos is also in rapid decline, use the West route [21] . Tracking birds from this population would be required to confirm this. Any colonization by birds using the West route may be quite recent, as before this study there was no evidence of birds from the United Kingdom using the West route [9] , as all ringing recoveries have been of birds apparently using the East route that is shared with birds from Scandinavia [22] . Alternatively, use of the West route could be a flexible response to delayed onset of autumn migration. Under this scenario, the route could potentially have arisen due to birds retracing the route of their spring migration. Finally, the West route could have arisen through reversal of the longitudinal component of the East route at a time when it conferred a selective advantage. Such an advantage could come from increased breeding opportunities arising from the later departure date of West birds, because the route is restricted to the geographical area (but not to those habitats) in which Reed Warblers, which continue breeding after male cuckoos have left the United Kingdom, are a major host. The fact that the two migration routes ultimately converge on the same wintering grounds is also very surprising as the use of different routes is usually a precursor to occupation of different wintering areas by different breeding populations [23] (a pattern known as migratory connectivity). The absence of migratory connectivity in this case is possibly a consequence of a restricted winter range forcing birds to occupy the same wintering area—that is, there are no possible equatorial or southern hemisphere wintering areas in West Africa due to the shape of the African continent. Alternatively, wintering location may be dictated by geographical variation in breeding phenology and by the timing of fuelling of spring migration at the wintering grounds [24] , resulting in birds from the same breeding area occupying the same wintering grounds. Why does the western route persist despite the increased mortality of birds using it? One possibility is that the conditions causing the increased mortality may have occurred only recently, or may not be consistent over longer timescales; thus, composition of breeding populations has not yet adjusted. Migratory birds are believed to have relatively inflexible annual migration programmes, implying that tracking of environmental variation may take some time [25] . Alternatively, mortality later in the annual cycle may offset the greater mortality up to this stage but in such a scenario, it is unlikely to be that there would be an association between route use and population change. There was no difference in survival between birds migrating via the two routes during the remainder of their southward migration in Africa ( Fig. 2 ), nor on the return migration from the Central African wintering grounds to the United Kingdom, although sample sizes were small for the latter. As there is no difference in where birds using the two routes spent the midwinter period ( Table 1 , Fig. 2a ), when they arrived there ( Table 1 ) or in the spring migration routes they used ( Fig. 2b ), they are likely to be exposed to similar pressures during the rest of their annual cycle. Previous work has demonstrated that constraints on the timing of spring migration can cause population declines in long-distance migratory birds [3] , [26] , via effects on reproductive productivity [3] . There has been mixed evidence of this for European Common Cuckoo populations [27] , [28] —future work needs to address the issue of whether there are constraints on the timing of spring migration that could cause a mismatch with breeding resource availability (including host nests in this case) in UK cuckoos. The results presented here, however, demonstrate that conditions during migration can also influence population dynamics of long-distance migrants via effects on survival and emphasize the need for a full annual cycle approach to understanding migratory life cycles [29] . Consequently, understanding variability in migratory behaviour and performance may be vital when attempting to understand population changes of these species. This may help to identify critical areas where stopover quality has declined and to predict the response of species to future climate change, allowing prioritization of conservation resources [30] . Further advances in the miniaturization of real-time tracking devices [31] should therefore result in the provision of extremely valuable information for the pressing concern of migratory land-bird conservation [1] , [4] , [5] , [30] , [32] , as well as the provision of important opportunities for raising awareness of these declines among the public [14] . Tagging and tracking Forty-seven adult male (second calendar year and older) Common Cuckoos Cuculus canorus canorus were tagged in Britain between 2011 and 2014, in nine geographically well-spread areas. These areas contrasted in recent local cuckoo breeding population change according to two independent data sets and represented a range of habitat types and therefore distinct communities of cuckoo hosts ( Supplementary Tables 1 and 2 ). The tagging was licensed by the Special Marks Technical Panel operating on behalf of the British Trust for Ornithology and the UK Government’s Home Office, and was carried out in accordance with their ethical guidelines. Birds were caught using mist-netting, sound lures (recordings of male and female cuckoo vocalizations) and a dummy (stuffed female Common Cuckoo) placed on a pole. Each individual was fitted with a PTT-100 from Microwave Telemetry weighing <5 g as a backpack using 2 mm diameter flat-braided nylon cord [22] . No birds weighing <115 g were tagged and the tags weighed 3.8–4.2% of the birds’ body weight on tagging. Each tag was programmed for a transmission duty cycle of 10 h on and 48 h off, to allow the battery to charge via the solar panel. With the exceptions of PTTs 115,586, 115,590, 115,599 and 121,791, tags deployed from 2013 were additionally programmed to transmit whenever the battery was close to fully charged but otherwise adhered to the scheduled duty cycle, providing extra positions when weather conditions were favourable. Satellite data Locations of the PTTs were obtained from the ARGOS system [33] . All data were Kalman filtered before locations being received, with the exception of data received before May 2012 from the five PTTs deployed in 2011. Mirror image locations were removed using the Douglas filter facility in Movebank and checked visually. These sometimes occurred even with Kalman filtering for the first location after the bird had moved a considerable distance from its previous position, but were easily identified based on subsequent locations. Analysis was carried out using a data set produced by selecting the best-quality location per duty cycle using Movebank method 1 (based on location class, error radii and number of messages), from a pool including locations for which the reliability could be assessed (classes 1, 2 and 3) and all other locations passing a plausibility filter based on speed-on movement or mutual validation via proximity (Movebank Douglas filter options: Method DAR; keeplc=1, mxred=10, minrate=120, ratecoef=25, minoffh=11 and rankmeth=1). Mortality All birds from which transmissions were lost were initially assumed to have died. Some studies [7] have been able to prove bird death in some instances through additional observations such as finding the corpse using final GPS coordinates but this is not possible here due to the lower accuracy of Doppler PTTs. As tagged birds are not colour marked and are rarely seen in the field, proving tag failure through field observations of birds after tracking has ceased is not possible. Some cases of tag failure are therefore likely to be included in the mortality rates for each route. Battery degradation through prolonged habitat-mediated shading resulting in charge depletion is the most probable cause of tag failure according to the manufacturer. It is not clear how probable is this during deployment as the tag enters ‘sleep’ mode requiring minimal power to protect the battery when the charge drops below a threshold. Background rates of tag failure in the absence of shading are estimated to be very low, around 1% in the initial 12 months after deployment (Paul Howey, Microwave Telemetry Inc., personal communication). Although rates of failure are unlikely to differ between the two routes at any point of the annual cycle, the greater chance of poor tag charge leading to loss of contact with a bird in the forest zone south of 6°N, where canopy cover is higher, means it could disproportionately affect apparent survival of birds after the Sahara crossing. Apparent survival was therefore calculated (1) up to completion of the Sahara crossing, (2) from that point until arrival at the stopover location of minimum latitude and (3) from there until arrival back in the United Kingdom. This was to prevent any tag failures during the second period differentially impacting apparent survival of birds from the route with higher survival in earlier periods. In some cases, evidence in support of mortality comes from the following: (1) tag remaining stationary for a prolonged period, especially in inhospitable terrain (for example, open desert) or non-seasonal locations (for example, throughout into the winter in Europe); (2) data from the tag’s temperature sensor indicating that it is no longer being buffered from diurnal environmental fluctuations by the bird’s body temperature. In both cases, the caveat is that the tag could have become detached from the live bird but this is extremely unlikely with the harness design used. In almost all cases in which contact with a tag is permanently lost (even when, for example, temperature information already indicates that the bird is dead), there is a short period where charge lowers, presumably due to the tag resting in a position where limited sunlight is reaching the solar panels. Longer periods of declining charge could, however, indicate technical failure of the tag. To account for the cases where lost contact is most likely to be indicative of tag technical failure, we therefore repeated the analysis excluding those instances where no further locations were received after a prolonged period of declining tag charge and there was no evidence in support of mortality before this. This resulted in the exclusion of two cases (one West and one East) from the stage up to completion of the Sahara crossing and one case (East) for the stage between completion of the Sahara crossing and arrival at the minimum latitude stopover/position occupied at midwinter. Remaining cases were those where there was either evidence that the bird had died or when contact was lost after no or only a short period of low or declining battery charge. Migration metrics Southwards migration routes and stopover areas were identified using all transmission either until transmissions stopped or until each bird reached its most southerly stopover (see below for definition of stopover), which was usually also the position occupied at mid-winter. After excluding journeys by five birds, which were lost to tracking before they reached southern Europe, 56 journeys by all birds were classified into either West or East migrating groups based on whether they left Europe via either Iberia or from Italy and eastwards. Individuals that were lost to tracking in southern Europe were classified according to the longitude of their final stopover location, as at this latitude the distributions of East and West birds that were tracked into Africa were discontinuous with the exception of one outlying bird and none of the birds classified by this method was close to the overlap. Stopovers were defined as periods when best locations from two or more consecutive scheduled transmission periods were within 50 km of each other, meaning the minimum duration of stopovers considered is 3 days. Stopovers of this duration could be missed if the best locations from the relevant duty cycles were away from the stopover location, or if there were no reliable locations from one duty cycle. Stopover duration was calculated by assuming that a bird arrived on the first day and departed on the last day that it was detected at a stopover location and hence are minima. Tags often showed gradually depleting battery charge during a stopover but in most cases charged and began transmitting on exposure to sunlight when a bird moved to a new location. Exceptions were therefore made when no locations were received for one or more transmission cycles before a bird was detected at a new location, in which case the bird was assumed to have remained at the previous stopover location until the day the last missed location was expected. Key migration events were defined as follows: departure from the breeding grounds was assumed to have occurred on the day before the first location more than 50 km away from it. Completion of the Sahara crossing was the day of the first location in the first stopover south of the Sahara. Completion of migration was the first day at the stopover with minimum latitude. Migration distance was the total distance moved between best locations per cycle, excluding movements within stopovers (that is, those <50 km), from departure until the completion of migration. Duration of migration was the number of days between the assumed day of departure and the first location at the minimum latitude stopover, which, in the majority of cases, was also the location occupied at midwinter. Migration speed was the total distance travelled divided by the duration. Number of stopovers was the number of stopover sites occupied before arrival at the most southerly location. Migration metrics were calculated: (a) to arrival in the first stopover south of the Sahara, the major barrier crossed during migration; and (b) to arrival at the most southerly stopover area occupied, for all individuals that completed the relevant migrations. The direction of the Sahara crossing was calculated (a) by taking the average of the bearings from the previous best of duty cycle position to all locations during active migration, which fell in Africa north of 15° N, or to the most northerly position below 15° N if there were none to the north, excluding positions in the Atlas mountains and the adjacent coast as suitable stopover locations exist there and (b) by calculating the bearing between the final pre- and first post-Sahara crossing stopover. Statistical analyses Analyses were undertaken using GLMMs in Proc Glimmix in SAS 9.2. Relationships between routes in migration metrics and apparent survival were modelled as a function of migration direction using Gaussian and binomial response distributions, respectively. Year and individual*region (‘region’ being tagging area) were initially included as random factors to account for dependencies with year and tagging area, and pseudo-replication due to the inclusion of repeated journeys from the same individual. Random factors were removed if their covariance parameter was zero. The LSMeans function was used to output estimates of each variable for each route. Differences in key stopover and wintering locations were additionally modelled using average latitude, average longitude and latitude*longitude as predictor variables with route as a binomial response variable. Results presented are marginal effects for the model with lowest pseudo-akaike information criteria (AIC). Models for the first stopover after the Sahara crossing failed to converge so the latitude and longitude for this stopover were tested separately. Local breeding population change around each tagging location was calculated by buffering all 10 km UK national grid squares in which a cuckoo was trapped for tagging by two 10 km 2 (that is, producing a minimum of 50 km 2 centred on a 10 km in which a cuckoo was tagged) and averaging population changes across all selected 10 km 2 for each of the nine tagging localities. Indexes of population change for each 10 km 2 were available from two completely independent data sets: the Bird Atlas 2007–11 (ref. 15 ) and the BTO/RSPB/JNCC BBS [16] . For the Bird Atlas, change in abundance was the standardized arithmetic difference between the abundance in 1988–91 and 2008–11. Abundance was calculated as the proportion of surveyed 2 km Atlas squares (39,936 were surveyed in 1988–91 and 45,374 in 2007–11 across Britain and Ireland) falling in each 10 km that were occupied by cuckoos [15] . For BBS, abundance for each 1 km 2 was produced by modelling counts from surveyed 1 km 2 for 1994–96 and 2007–09 (between 1,501 and 3,018 survey squares each year) with respect to landcover, northing, easting, elevation and including a smoothing term in a GAM [16] . The results were them condensed to give abundance values at the 10 km 2 level and change was calculated as the estimated abundance index for 2007–09 minus the estimated abundance index in 1994–96. The two population change data sets are completely independent. The change index from the Atlas is, however, far more robust and spatially precise than the change from BBS, because it is based on an order-of-magnitude greater number of data points, with no interpolation or spatial smoothing such as used in the BBS data set, with more field survey effort underlying each data point. As such, it is far more appropriate to determine local population changes. Relationships between local breeding population change and migration direction were then modelled using events/trials logistics regressions with each tagging locality as a case, number migrating east as the numerator and total number tagged as the denominator on the dependent variable and average breeding population change index as the explanatory variable. Each bird is therefore represented as a single migration direction, irrespective of how many journeys it was tracked over. In the single instance in which a bird used different routes on consecutive journeys (see Supplementary Fig. 1 ) a classification of 0.5 was given to each route. A habitat variable classifying each tagging locality as upland or lowland was subsequently added to test whether relationships remained when controlling for this division. The altitudinal distribution of vegetation types differs greatly across the tagging locations due to geographical climatic variation; thus, upland was defined as areas in which the surrounding landscapes were predominantly mires, wet heaths and acid grassland. Data availability The authors declare that the data supporting the findings of this study are available in Supplementary Tables 1–6 . How to cite this article: Hewson, C. M. et al . Population decline is linked to migration route in the Common Cuckoo. Nat. Commun. 7:12296 doi: 10.1038/ncomms12296 (2016).